Patterning symmetry in the rational design of colloidal crystals Colloidal particles have the right size to form ordered structures with periodicities comparable to the wavelength of visible light. The tantalizing colours of precious opals and the colour of some species of birds are examples of polycrystalline colloidal structures found in nature. Driven by the demands of several emergent technologies, efforts have been made to develop efficient, self-assembly-based methodologies for generating colloidal single crystals with well-defined morphologies. Somewhat unfortunately, these efforts are often frustrated by the formation of structures lacking long-range order. Here we show that the rational design of patch shape and symmetry can drive patchy colloids to crystallize in a single, selected morphology by structurally eliminating undesired polymorphs. We provide a proof of this concept through the numerical investigation of triblock Janus colloids. One particular choice of patch symmetry yields, via spontaneous crystallization, a pure tetrastack lattice, a structure with attractive photonic properties, whereas another one results in a colloidal clathrate-like structure, in both cases without any interfering polymorphs. In contrast to typical atomic and molecular systems, colloidal particles interact via effective potentials characterized by excluded volume and an interaction range usually much smaller than the particle size. As a consequence, the potential energy contribution to the crystal stability is controlled by the location of nearest neighbours, so that crystals with similar local environments are stabilized energetically in a comparable way. The canonical case of such behaviour are the crystals formed by hard spheres, where the free energy of the face-centred cubic (FCC) and the hexagonal close packed (HCP) lattices, two structures differing only for the stacking of adjacent hexagonal planes ( Fig. 1a–c ), are the same to within a small fraction of the thermal energy [1] , [2] . Indeed, hard-sphere colloids crystallize into coexisting regions of face-centred cubic and hexagonal closed-packed structures both in simulations [3] and experiments [4] . An equally relevant case is provided by the cubic and hexagonal morphologies of the diamond, different only in the way that planes are stacked along one direction ( Fig. 1d–f ). The similarity in free energy between such closely related morphologies has profound consequences on the formation of pure crystals: it becomes extremely difficult to avoid stacking hybrids of the two structures in the crystallization process [3] , [5] . This problem is particularly relevant for photonic applications, where the long-range order of the structure is crucial in determining its optical properties. It is therefore unfortunate that the structures with the most desirable transmission properties, that is, diamond [6] and tetrastack [7] ( Fig. 1g–i ), both suffer from the deleterious possibility of forming stacking hybrids with a structure of different global symmetry, namely hexagonal as opposed to cubic. 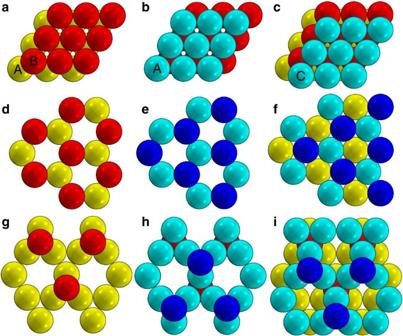Figure 1: Stacking-fault prone crystalline structures. Visualization of the layer-by-layer build-up of the face centred cubic and of the hexagonal close-packed (FCC/HCP, top row), of the cubic and hexagonal diamond (DC/DH, middle row) and of the cubic and hexagonal tetrastack (CT/HT, bottom row) crystalline structures. The cubic and hexagonal structures arise from different orientations of adjacent planes. (a) Top view of two adjacent triangular planes. The successive plane can be placed in two different ways, exactly on top of the first (b, ABAB stacking, originating, if repeated, the HCP structure) or shifted (c, ABC stacking, originating the FCC). Hybrid structures can be generated by arbitrary sequences of A, B and C planes. (d) Top view of the (undulated) plane that can be stacked to form hexagonal (e) or cubic (f) diamond. In the DH case, particles on the next layer are sitting exactly on top of the previous layer. In the DC case, half of the particles on the top plane superimpose to the holes of the bottom plane. Again, hybrid structures can be generated by arbitrary stacking. (g) Arrangement of (a dense and a dilute) two-layer structure that can be stacked to create a hexagonal (h) or cubic (i) tetrastack. In the HT case, particles on the dense (red and cyan) layers are sitting exactly on top of the previous dense layer, whereas in the CT, successive dense layers are shifted by a particle diameter. Particles on the dense layers are all in staggered configurations, whereas particles in the dilute layers (red and blue) are staggered in CT and eclipsed in HT. Figure 1: Stacking-fault prone crystalline structures. Visualization of the layer-by-layer build-up of the face centred cubic and of the hexagonal close-packed (FCC/HCP, top row), of the cubic and hexagonal diamond (DC/DH, middle row) and of the cubic and hexagonal tetrastack (CT/HT, bottom row) crystalline structures. The cubic and hexagonal structures arise from different orientations of adjacent planes. ( a ) Top view of two adjacent triangular planes. The successive plane can be placed in two different ways, exactly on top of the first ( b , ABAB stacking, originating, if repeated, the HCP structure) or shifted ( c , ABC stacking, originating the FCC). Hybrid structures can be generated by arbitrary sequences of A, B and C planes. ( d ) Top view of the (undulated) plane that can be stacked to form hexagonal ( e ) or cubic ( f ) diamond. In the DH case, particles on the next layer are sitting exactly on top of the previous layer. In the DC case, half of the particles on the top plane superimpose to the holes of the bottom plane. Again, hybrid structures can be generated by arbitrary stacking. ( g ) Arrangement of (a dense and a dilute) two-layer structure that can be stacked to create a hexagonal ( h ) or cubic ( i ) tetrastack. In the HT case, particles on the dense (red and cyan) layers are sitting exactly on top of the previous dense layer, whereas in the CT, successive dense layers are shifted by a particle diameter. Particles on the dense layers are all in staggered configurations, whereas particles in the dilute layers (red and blue) are staggered in CT and eclipsed in HT. Full size image Inspired by recent developments in the synthesis and understanding of patchy colloids [8] , [9] , [10] , [11] , [12] , we introduce here a new concept in colloidal design that we call patterning symmetry, with the aim of structurally suppressing the undesired competing crystal and favouring the self-assembly of the desired structure. We apply our idea, as an example, to the technologically relevant case of the self-assembly of a cubic tetrastack (CT) and a colloidal clathrate lattice. The CT is a close relative of the cubic diamond, as it can be generated by placing a particle halfway between adjacent sites of a cubic diamond lattice. As a result, each particle has six neighbours ( Fig. 1i ), three above it and three below it, in a staggered configuration. The naive design of patchy particles that self-assemble into a tetrastack lattice would consist of spheres decorated with six small patches in a geometry matching the distribution of the contacts observed in the target lattice. However, patterning a particle's surface in such a sophisticated geometry is beyond routine experimental protocols. Recent experimental work by Chen et al . [13] investigating the self-assembly into a two-dimensional (2D) Kagome lattice has shown that control on the structure can be gained by using only two circular patches, but limiting the number of bonded neighbours via a proper selection of the patch width. As discussed later, we attempted to exploit this idea for the self-assembly of three-dimensional (3D) crystals but found that Janus particles with two circular patches allowing for three contacts each spontaneously form only mixed morphologies, similarly to hard-sphere colloids. Assembly in 3D apparently requires more than careful control over the number of neighbours if more than one lattice is compatible with the local arrangement imposed by the patch placement ( Fig. 1 ). The novelty of our work is that the use of the patch symmetry circumvents this problem, and yields different single crystals depending on the patch orientation. Phase diagram of triblock Janus particles We start by documenting the formation of stacking hybrids in the case of circular patches triblock Janus particles. We model them via the two-patch Kern–Frenkel [14] potential, selecting the patch width so that each patch can form at most three contacts. This model has already been validated against experiments and shown to successfully describe the thermodynamics and self-assembly of triblock Janus particles in 2D [15] , as well as the fluid state in 3D [16] . Furthermore, the one-patch analogue [17] has been studied as a model for two-block Janus particles [18] . Two-patch particles in three dimension can form several crystal structures in which each patch is involved in three contacts. Besides the close-packed structures, which can be generated also with spherically interacting colloids, these particles allow for the formation of open lattices. The tetrastack crystal, which can be seen as the three-dimensional extension of the two-dimensional Kagome lattice [13] , is indeed compatible with such patch arrangement. We evaluate first the free energy of the different crystal structures via the methodology described in ref. 19 and tailored to patchy models in refs 20 , 21 , 22 (Methods). At low temperature T , crystal stability is controlled by the potential energy and thus only fully bonded structures appear in the phase diagram. The expected competition between crystals with different symmetries clearly manifests itself in the phase diagram ( Fig. 2 ). Indeed, the fully bonded structures include at low densities both the open CT and its hexagonal counterpart, which we shall call hexagonal tetrastack (HT), and at high densities the FCC and HCP crystals. Just like the CT can be obtained from the cubic diamond by placing a particle halfway in between the neighbouring lattice points, the HT can be obtained in the same way by starting from the hexagonal diamond (lonsdaleite). Other possible fully bonded open crystal structures (clathrates-like, see later) have been found to be only metastable and do not appear on the equilibrium phase diagram. Within our numerical precision (≈0.02 k B T ), the fully bonded cubic and hexagonal structures have the same chemical potential at all the state points investigated. Hence, the high-density FCC and HCP and the low-density CT and HT share the same stability region in the phase diagram of particles with circular patches ( Fig. 2 ). 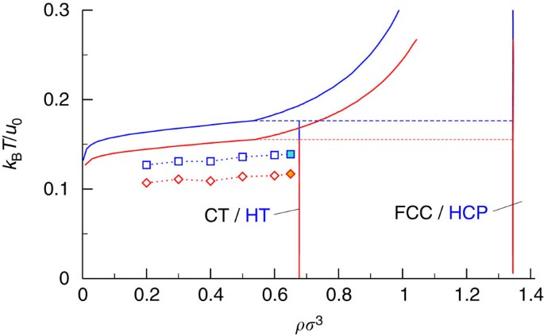Figure 2: Low-temperature phase diagrams for particles with circular and staggered triangular patches. The density range in which crystals are stable is the same for the two models. Black labels refer to both models while blue labels refer only to particles with circular patches. Squares indicate the homogeneous nucleation line of the hybrid CT/HT crystal fromNVTsimulations of particles with circular patches. Diamonds mark the homogeneous nucleation line for particles with triangular patches, resulting in a pure cubic tetrastack. The filled points are studied in more detail inFig. 2. For both models, theTat which nucleation is observed is larger than one tenth of the interaction strength, aTwhich allows for thermal breaking and reforming of the contacts, both in simulations and in experiments. Figure 2: Low-temperature phase diagrams for particles with circular and staggered triangular patches. The density range in which crystals are stable is the same for the two models. Black labels refer to both models while blue labels refer only to particles with circular patches. Squares indicate the homogeneous nucleation line of the hybrid CT/HT crystal from NVT simulations of particles with circular patches. Diamonds mark the homogeneous nucleation line for particles with triangular patches, resulting in a pure cubic tetrastack. The filled points are studied in more detail in Fig. 2 . For both models, the T at which nucleation is observed is larger than one tenth of the interaction strength, a T which allows for thermal breaking and reforming of the contacts, both in simulations and in experiments. Full size image Given their typical dimensions and timescales associated with their motion, colloidal particles may have difficulties in reaching equilibrium owing to the possible presence of kinetic traps. It is thus important to study whether the equilibrium phase diagram is of relevance for the present model or if the kinetic arrest associated with possible gel or glass transitions hampers the possibility of forming crystal phases. To address this issue, we perform several Monte Carlo simulations in metastable state points to detect the onset of crystallization and the nature of the resulting crystal. We discover that indeed kinetic traps are not present and that the investigated system easily crystallize. The line in the T – ρ plane along which crystallization is observed in simulation (the homogeneous nucleation line for our observation time and system size) is traced in Fig. 2 . Triblock Janus particles are very good crystal formers, as their nucleation T is sufficiently high to prevent locking into bonded configuration and significantly larger than the gel/glass T as well as than the gas–liquid phase separation T , a phenomenon that could interfere with the crystallization process. We thus perform Monte Carlo simulations of large systems under mild supercooling to observe the formation of a single crystal and analyse its structure. The analysis of the final configurations (see Methods and Supplementary Methods ) shows that the structure is a mixture of CT and HT layers. 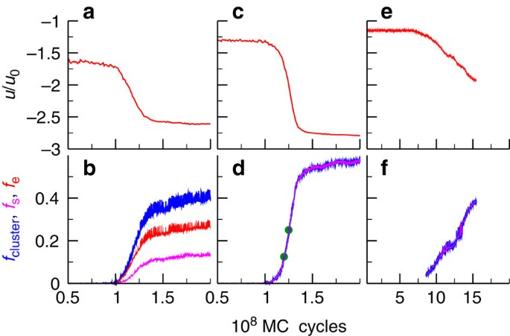Figure 3: Crystal nucleation kinetics for circular, staggered and eclipsed patches. Nucleation of the crystal from the fluid phase at ρσ3=0.65 in the NVT ensemble (N=4,000), just below the equilibrium ρ of the hexagonal and cubic tetrastack (see filled square and diamond inFig. 1, respectively for particles with circular (T=0.138) and staggered (T=0.117) patches). A clear jump in the energy per particle (that in our simple model is just half the number of contacts) as a function of Monte Carlo steps (a,c) marks the nucleation event. Analysis of the configurations confirms that a single crystal is growing (see text). Snapshot of the clusters corresponding to the circles indare reported inSupplementary Fig. S3and are available asSupplementary Datafor visual inspection. For both patch shapes, the nucleation is associated with an increase in the fractionfcluster(blue lines) of particles in the largest crystalline cluster (b,d).N·fclusteris the size of the growing cluster. But the fraction of eclipsedfe(red lines) and staggeredfs(magenta lines) particles, which are both in the largest cluster as well as have an eclipsed and staggered local geometry, is different in the two cases; for staggered triangular patches,fs=fclusterandfe=0, whereas for circular patches, bothfsandfeare a significant fraction, signalling the presence of stacking faults. The right column shows the crystallization of the clathrate-like structures for particles with eclipsed triangular patches atρ=0.5 andT=0.114. At this state point, more than one crystal cluster nucleates, so the energy jump is less sharp (panele). Inf, we report the fraction of crystalline particles in the system (that is, regardless of them being in the largest cluster or not); all of them are in eclipsed configurations, as dictated by the patch shape. Figure 3a,b reports the evolution of the potential energy and of the fraction of particles in the largest crystalline cluster. It also shows the fraction of particles in cubic and hexagonal local geometries (Methods). The growing crystal is a mixture of interconnected CT and HT local structures, confirming that the triblock Janus particles with circular patches, despite their ability to nucleate the open tetrastack structure, are not optimal candidates for self-assembling a pure crystal. Hence, as already known for the FCC/HCP [3] and the cubic and hexagonal diamond [5] , spontaneous crystallization results into a structure with no long-range order owing to the formation of stacking hybrids of the CT and HT polymorphs. Figure 3: Crystal nucleation kinetics for circular, staggered and eclipsed patches. Nucleation of the crystal from the fluid phase at ρ σ 3 =0.65 in the NVT ensemble ( N =4,000), just below the equilibrium ρ of the hexagonal and cubic tetrastack (see filled square and diamond in Fig. 1 , respectively for particles with circular ( T =0.138) and staggered ( T =0.117) patches). A clear jump in the energy per particle (that in our simple model is just half the number of contacts) as a function of Monte Carlo steps ( a , c ) marks the nucleation event. Analysis of the configurations confirms that a single crystal is growing (see text). Snapshot of the clusters corresponding to the circles in d are reported in Supplementary Fig. S3 and are available as Supplementary Data for visual inspection. For both patch shapes, the nucleation is associated with an increase in the fraction f cluster (blue lines) of particles in the largest crystalline cluster ( b , d ). N · f cluster is the size of the growing cluster. But the fraction of eclipsed f e (red lines) and staggered f s (magenta lines) particles, which are both in the largest cluster as well as have an eclipsed and staggered local geometry, is different in the two cases; for staggered triangular patches, f s = f cluster and f e =0, whereas for circular patches, both f s and f e are a significant fraction, signalling the presence of stacking faults. The right column shows the crystallization of the clathrate-like structures for particles with eclipsed triangular patches at ρ =0.5 and T =0.114. At this state point, more than one crystal cluster nucleates, so the energy jump is less sharp (panel e ). In f , we report the fraction of crystalline particles in the system (that is, regardless of them being in the largest cluster or not); all of them are in eclipsed configurations, as dictated by the patch shape. Full size image Implementing patterning symmetry In the 2D system investigated by Granick and co-workers, the rational design strategy encoded in the patch width has been successful in self-assembling the Kagome lattice [13] . Clearly, in the 3D case, our results show that one needs to go one step further in the rational design strategy, because more than one crystal is compatible with the first-neighbour arrangement imposed by the patches. As the interaction range is short, selection among the competing structures, which differ only at the level of third neighbours, cannot be achieved directly by modulation of the interaction potential. We then propose to resort to the patterning symmetry concept: select the local geometry acting on the patch shape to impose the relative arrangement of second neighbours (eclipsed in CT or staggered in HT, Fig. 4 ). Specifically, we propose to pattern the colloidal particles with two triangular patches oriented in a staggered geometry. Such asymmetric patterning, which is readily achievable within current synthesis methodologies [23] , [24] , only allows for staggered configurations ( Fig. 4 ) and thus forbids the formation of hexagonal structures. The phase diagram of particles with staggered triangular patches (modelled via a generalization of the Kern–Frenk potential as described in the Methods) is similar to that of the particles with circular patches, except that it does not include the two hexagonal crystals ( Fig. 2 ). The modified patch shape and particle symmetry completely removes the structural degeneracies and the possibility of forming stacking hybrids. This is the central idea of our work. 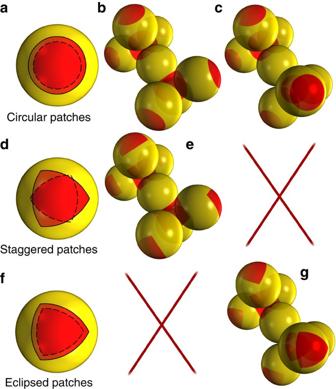Figure 4: The patterning symmetry concept. Triblock Janus particles with circular patches (a) can form fully bonded staggered (b) and eclipsed (c) configurations. Particles with staggered triangular patches (d) can only form fully bonded configurations in staggered geometry (e), while particles with eclipsed triangular patches (f) only form fully bonded eclipsed local arrangements (g). The choice of staggered triangular patches singles out the FCC and CT lattices, because these structures do not contain eclipsed local geometries. Similarly, colloidal clathrates are formed only by eclipsed local geometries and are thus selected by the choice of eclipsed triangular patches. Figure 4: The patterning symmetry concept. Triblock Janus particles with circular patches ( a ) can form fully bonded staggered ( b ) and eclipsed ( c ) configurations. Particles with staggered triangular patches ( d ) can only form fully bonded configurations in staggered geometry ( e ), while particles with eclipsed triangular patches ( f ) only form fully bonded eclipsed local arrangements ( g ). The choice of staggered triangular patches singles out the FCC and CT lattices, because these structures do not contain eclipsed local geometries. Similarly, colloidal clathrates are formed only by eclipsed local geometries and are thus selected by the choice of eclipsed triangular patches. Full size image To confirm that the triblock Janus particles patterned with staggered triangular patches crystallize in 3D into a CT, we investigate the nucleation process both in constant pressure and constant density simulations. The asymmetric patterning, beside removing global hexagonal ordering, also removes the local competition between the two arrangements facilitating the nucleation process. The resulting growing CT crystal clusters are very well defined and defect-free. The nucleation processes is visualized in Fig. 3c–d , showing that no eclipsed configurations are present in the nucleated structure. The lower symmetry of particles with triangular patches, however, comes at the expense of a decrease of the nucleation T , because of the lower number of orientations compatible with full bonding causing an extra entropic cost for crystallization. Still, nucleation takes place when the strength of the interaction is less than ten times the thermal energy, a condition that is within the experimentally accessible values. Indeed, experimental estimates provided by Chen et. al. [13] suggest a value of u 0 of the order of 10 k B T . It is worth pointing out that this T allows for contact rearrangement and, thus, annealing of structural defects in the nucleated structure. Robustness to fabrication defects To prove that our strategy is robust to imperfections in the patch placement/position inevitably arising from the fabrication process, we have repeated our calculations introducing some degree of disorder in both the patch size and in the patch position (see Methods and Supplementary Figs S1 and S2 ). As shown in the results reported in Supplementary Table S1 , we find that, in all cases, the total number of crystal particles n c is comparable with the size of the largest crystalline cluster, and hence the nucleation process involves one single nucleus. The observed crystal structure is in all cases the cubic tetrastack, providing strong evidence that disorder in the patch width does not hinder its formation. This confirms that crystallization in a pure cubic tetrastack structure occurs for a patch size disorder comparable with what estimated in experiments [13] . We also repeat our study with a potential with a smooth attraction, again with no significant change in the final outcome (see Methods and Supplementary Figs S4 and S5 ). Eclipsed patches The patterning symmetry concept is of wide applicability. The choice of the eclipsed patch arrangement not only allows to select between CT and HT, but it also discriminates FCC from HCP. As an additional interesting case, one can pattern two eclipsed triangles on the particle's poles, as against the case of two staggered triangles considered above. Here one can selectively eliminate from the phase diagram of particles with circular patches both the cubic and the hexagonal structures, because they all require some staggered configurations. The low T phase diagram of particles with eclipsed triangular patches ( Fig. 4f ) can display only fully bonded solids formed by 100% particles in eclipsed local geometries. The sI and sII [25] clathrates, found in hydrates such as Cl 2 in solid H 2 O (refs 26 , 27 ) satisfy this requirement. These structures, rich in pentagonal rings, are essentially crystals of empty icosidodecahedra, linked by bridge particles. A representation of the icosidodecahedron is shown in Fig. 5 . The same transformation of the diamond into a tetrastack, applied to the sI and sII tetrahedral structures, generates six-coordinated, fully eclipsed lattices with large unit cells (68 and 92 particles, respectively). In our simulations, we have observed the spontaneous self-assembly of the eclipsed triangular patches in these clathrate structures at density and temperature comparable to those of the crystallization of particles with triangular patches, albeit with slower kinetics consistently with the complexity of the large unit cell. ( Fig. 3e,f ). 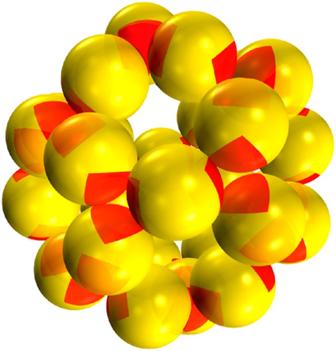Figure 5: Clathrate-like structure with eclipsed patches. Representation of an icosidodecahedron, the basic unit of the clathrate lattices, composed of eclipsed triblock Janus particles. Figure 5: Clathrate-like structure with eclipsed patches. Representation of an icosidodecahedron, the basic unit of the clathrate lattices, composed of eclipsed triblock Janus particles. Full size image In summary, we have introduced a novel key element in the rational design of patchy colloids. We show that we can self-assemble a highly relevant 3D complex collective structure by using simple elementary particle-building blocks, within the reach of today's experimental capabilities [13] , [23] , [24] . The proposed patterning symmetry strategy, which imposes the second-neighbour arrangement through control over patch orientation, removes the competition between wanted and unwanted crystal structures with similar free energies, circumventing a common problem in the crystallization of colloids with short-range interaction potential. Patterning symmetry also improves the selectivity of the fully bonded structures, stabilizing unconventional lattices, such as the colloidal clathrates formed by eclipsed triangular patches. Finally, the selection of the local geometry cleans up the self-assembly process, eliminating competing low-energy local geometries incompatible with long-range order and reducing the probability that the system becomes trapped into a glassy state. In the specific example reported, no bottlenecks are present along the crystallization path towards the spontaneous formation of the CT or the clathrate crystal. Because the experimental implementation of the patterning symmetry rational design seems to be within the reach of present-day technology [13] , [23] , [24] , our work paves the way for the experimental realization of open colloidal single crystals. Interaction Potentials Circular patches: we model the triblock patchy particles via the Kern–Frenkel potential [14] . Each particle is described as a hard sphere of diameter σ whose surface is decorated with two attractive patches on the poles ( Fig. 4a ). In this model, the patches can be seen as the intersection of the particle's surface and a cone of aperture θ originating at the particle's centre and aligned along a (unit) vector , where n =1,2. Here and in the particle's reference frame. By defining as the position of the centre of particle i , and , the pair interaction is: In this work, cos θ =0.77, to allow for a maximum of three bonds per patch. Following experimental estimates [13] , we model the very short-range nature of the hydrophobic attraction choosing δ =0.03 σ. Triangular patches: to model particles with staggered triangular patches, we extend the Kern–Frenkel model. We define six virtual patches of width cos θ =0.427, to guarantee a maximum of three bonds per patch, centred on the vectors (in the particle reference frame) The overlap of the virtual patches centred on , and and the overlap of , and identify two triangularly shaped patches on opposite poles. As in the Kern–Frenkel model, two particles are bonded if σ< r ij <σ+ δ and if the vector r ij crosses one patch on each particle. Particles with eclipsed triangular patches ( Fig. 4g ) can be obtained by changing the vectors , and to: Simulation methods We perform standard Monte Carlo simulation of a system of N =4,000 particles in the canonical (NVT) and isothermal-isobaric (NPT) ensembles, where the three sides of the simulation box are allowed to change independently. A Monte Carlo step is defined as N attempts to randomly translate and rotate a randomly chosen particle. Free energy computations are carried out following the methodology outlined in ref. 19 . We perform thermodynamic integration to compute the (Gibbs) free energy of the fluid and a Frenkel–Ladd [28] approach to compute the free energy of solid phases. The orientational degrees of freedom in the Frenkel–Ladd procedure are treated with a referece hamiltonian chosen according to the particles symmetry, namely D ∞h for particles with circular patches and D 3D for particles with staggered triangular patches. In performing thermodynamic integration, no first-order phase transition lines (for example, the gas-liquid transition) must be crossed along the integrations path. Our calculations are based on thermodynamic integration along paths that are designed (and checked a posteriori ) to be free of first order transitions. The gas–liquid phase separation does not appear in the phase diagram of the model, because it is significantly depressed with respect to the homogeneous nucleation line. Indeed, even when the range of the attraction is of the order of 50%, the case extensively studied in ref. 16 , the gas–liquid becomes metastable below coverage 30%. In the circular patch model we have investigated the coverage is 23%. The reduction of the radial interaction range (only 3% in the present study) adds on this, making even harder to approach in a metastable equilibrium condition the gas–liquid coexistence. Modelling of the imperfections A straightforward way to model fabrication imperfections in the patches is to introduce disorder in the potential parameters controlling their size and position (equation 1). Suitable parameters to be perturbed are the positions of the virtual patches ( ) and their widths ( ). To model disorder in the patch width, we vary the value of so that each virtual patch (whose overlap generates the patch shape) has a different width. All virtual patches in the system are independently modified ( Fig. 6 ). The specific values of are drawn from a Gaussian distribution with mean , the value studied for the model discussed in the main text, and s.d. σ θ . We focus on two different values σ θ =0.02 and 0.04, which generate a typical error in the patch width of 2.5 and 5 degrees, respectively. 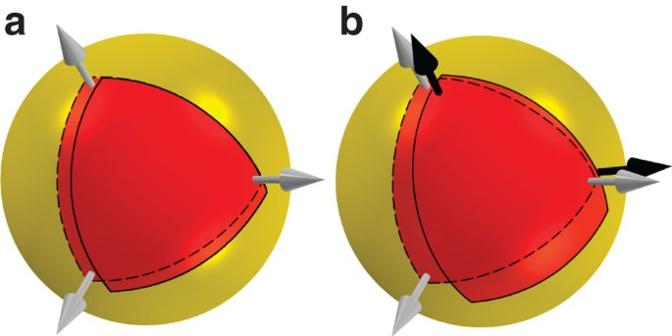Figure 6: Modeling disorder in the patch width and position. In (a), the three values ofhave been perturbed by 2σθ,−2σθand 0 withσθ=0.04. In (b), thevalues have been perturbed by δαk,i=δβk,i=2σp,−2σpwithσp=0.04. The dashed line indicates the corresponding ideal patch case. Figure 6: Modeling disorder in the patch width and position. In ( a ), the three values of have been perturbed by 2 σ θ ,−2 σ θ and 0 with σ θ =0.04. In ( b ), the values have been perturbed by δα k , i =δβ k , i =2 σ p ,−2 σ p with σ p =0.04. The dashed line indicates the corresponding ideal patch case. Full size image We have also studied how imperfections in the patch positions can affect crystallization. In this case, imperfections have been modelled by perturbing the (virtual) patch positions of equations (2), (3), (4), (5), (6), (7) in the main text. In this context, it is useful to rewrite equations (2), (3), (4), (5), (6), (7) as follows: with with for k =1, 2, 3 and for k =4, 5, 6, β 0, k =[0,2π/3,4π/3,π,π/3,5π/3] for k =[1...6]. In the ideal model, δα k , i =δβ k , i =0 for all ( i , k ) and equation 11 reduces to equations (2), (3), (4), (5), (6), (7). The perturbations δα k , i and δβ k , i have the effect of moving the centre of each virtual patch on the particle's surface, distorting the shape of the triangular patch. We have used values of δα k , i and δβ k , i drawn from a Gaussian distribution with 0 mean and σ p =0.02 and 0.04. These values correspond to a variance in the average patch displacement from the ideal position of about 1 and 2 degrees. A comparison between the idealized patch shape studied in the main text and a typical perturbed shapes is shown in Fig. 6 (right). Crystallization To calculate the largest crystalline cluster, we start by classifying a particle as crystalline if it has six bonded neighbours and no extra non-bonded neighbours within σ + δ . A crystalline link connects two crystalline particles if they have negative interaction energy. The connections in the link set are then used to partition particles into crystal clusters and evaluate the fraction of particles in the largest cluster f cluster ( Fig. 3 ). Investigation with other order parameters [29] yields the same results. To investigate the symmetry of the crystal and the possible presence of stacking faults, we further classify particles belonging to the largest crystalline cluster into eclipsed or staggered according to the geometric arrangement of their six neighbours (undefined arrangements are extremely rare in crystalline clusters). This allows us to evaluate the fraction of eclipsed ( f e ) and staggered ( f s ) particles, in the largest crystalline cluster (normalized to N ). In cubic structures f e =0 and f s = f cluster whereas in hexagonal lattices f e =0.25 f cluster and f s =0.75 f cluster . In clathrate structures, f e = f cluster and f s =0. Other values indicate the presence of stacking faults. How to cite this article: Romano, F & Sciortino, F, Patterning symmetry in the rational design of colloidal crystals. Nat. Commun. 3:975 doi: 10.1038/ncomms1968 (2012).